Novel loci affecting iron homeostasis and their effects in individuals at risk for hemochromatosis Variation in body iron is associated with or causes diseases, including anaemia and iron overload. Here, we analyse genetic association data on biochemical markers of iron status from 11 European-population studies, with replication in eight additional cohorts (total up to 48,972 subjects). We find 11 genome-wide-significant ( P <5 × 10 −8 ) loci, some including known iron-related genes ( HFE, SLC40A1, TF, TFR2, TFRC, TMPRSS6 ) and others novel ( ABO, ARNTL , FADS2, NAT2 , TEX14 ). SNPs at ARNTL, TF , and TFR2 affect iron markers in HFE C282Y homozygotes at risk for hemochromatosis. There is substantial overlap between our iron loci and loci affecting erythrocyte and lipid phenotypes. These results will facilitate investigation of the roles of iron in disease. Absorption, transport and storage of iron are tightly regulated, as expected for an element, which is both essential and potentially toxic. Iron deficiency is the leading cause of anaemia [1] , and it also compromises immune function [2] and cognitive development [3] . Iron overload damages the liver and other organs in hereditary hemochromatosis [4] , and in thalassaemia patients with both transfusion and non-transfusion-related iron accumulation [5] . Excess iron has harmful effects in chronic liver diseases caused by excessive alcohol, obesity or viruses [6] . There is evidence for involvement of iron in neurodegenerative diseases [7] , [8] , [9] and in Type 2 diabetes [10] , [11] . Variation in transferrin saturation, a biomarker of iron status, has been associated with mortality in patients with diabetes [12] and in the general population [13] . All these associations between iron and either clinical disease or pathological processes make it important to understand the causes of variation in iron status. Importantly, information on genetic causes of variation can be used in Mendelian randomization studies to test whether variation in iron status is a cause or consequence of disease [14] , [15] . We have used biomarkers of iron status (serum iron, transferrin, transferrin saturation and ferritin), which are commonly used clinically and readily measurable in thousands of individuals, and carried out a meta-analysis of human genome-wide association study (GWAS) data from 11 discovery and eight replication cohorts. These phenotypes show significant heritability in normal adults [16] , [17] , and previous population-based studies have identified relevant single-nucleotide polymorphisms (SNPs) and gene loci ( HFE, TF, TFR2 and TMPRSS6 (refs 18 , 19 )) for iron status biomarkers. HFE and TMPRSS6 have also been shown to affect red cell count, haemoglobin and erythrocyte indices [20] , most likely by affecting iron availability [20] , [21] , [22] . Our aims were to identify additional loci affecting markers of iron status in the general population and to relate the significant loci to information on gene expression to identify relevant genes. We also made an initial assessment of whether any such loci affect iron status in HFE C282Y homozygotes, who are at genetic risk of HFE -related iron overload (hereditary hemochromatosis type 1, OMIM #235200). Combination of results from discovery and replication stages of our analysis shows significant effects on one or more of the iron biomarkers at 11 loci. Those primarily affecting serum iron and transferrin saturation include, or are close to, genes whose products have recognized roles in iron homeostasis; HFE (the haemochromatosis gene) , TMPRSS6 (transmembrane protease, serine 6) and TFR2 (transferrin receptor 2). Those mainly affecting serum transferrin, apart from the TF (transferrin) gene itself and TFRC (transferrin receptor), and those mainly affecting ferritin (apart from SLC40A1 , solute carrier family 40 (iron-regulated transporter), member 1) are unexpected. There is a significant overlap between the genes or loci affecting iron biomarkers and those known to affect erythrocyte numbers or size, which is reasonable given the importance of iron for erythropoesis. We also find significant overlap between genes or loci affecting iron biomarkers and known loci affecting plasma lipids or lipoproteins, showing an unexplained link between these areas of metabolism. 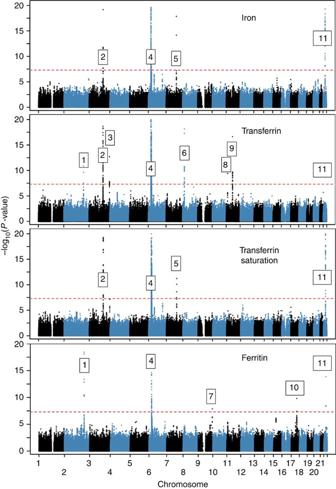Figure 1: Manhattan plots for the associations between SNPs and iron status (serum iron, transferrin, transferrin saturation and ferritin). The −log(p) values are from inverse-variance-weighted meta-analysis of the combined Discovery+Replication datasets for SNPs taken forward for replication, otherwise from the Discovery datasets only. Genes are assigned to the loci as follows: 1SLC40A1; 2TF; 3TFRC; 4HFE; 5TFR2; 6NAT2; 7ABO; 8ARNTL; 9FADS2; 10TEX14; 11TMPRSS6. Note that theyaxis for −log(P) values is truncated at 20. SNP and gene associations The combination of allelic association data from 11 discovery and eight replication cohorts ( Supplementary Tables 1–3 ) showed 11 loci with significant effects on one or more of the iron-related phenotypes ( Table 1 , Fig. 1 , Supplementary Figs 1 and 2 , Supplementary Table 4 ). Four of these ( HFE, TF, TFR2 , TMPRSS6 ) were previously known to affect iron biomarker variation in the general population [18] , [19] . Genes at two newly significant loci, SLC40A1 , which codes for the cellular iron exporter ferroportin and TFRC , which codes for the iron importer transferrin receptor 1, are known to be important for cellular iron homeostasis [23] . The other five loci (chromosome 8 at 18.3 Mbp, nearest gene NAT2 ; chromosome 9 at 136.2 Mbp, nearest gene ABO ; chromosome 11 at 13.4 Mbp, nearest gene ARNTL ; chromosome 11 at 61.6 Mbp, nearest gene FADS2 ; chromosome 17 at 54.1 Mbp, nearest gene TEX14 ) were not previously known to affect any of these phenotypes. These affect either transferrin ( NAT2, ARNTL , FADS2 ) or ferritin ( ABO, TEX14 ). Table 1 Results from discovery, discovery and replication, and conditional analyses. Full size table Figure 1: Manhattan plots for the associations between SNPs and iron status (serum iron, transferrin, transferrin saturation and ferritin). The −log(p) values are from inverse-variance-weighted meta-analysis of the combined Discovery+Replication datasets for SNPs taken forward for replication, otherwise from the Discovery datasets only. Genes are assigned to the loci as follows: 1 SLC40A1 ; 2 TF ; 3 TFRC ; 4 HFE ; 5 TFR2 ; 6 NAT2 ; 7 ABO ; 8 ARNTL ; 9 FADS2 ; 10 TEX14 ; 11 TMPRSS6 . Note that the y axis for −log( P ) values is truncated at 20. Full size image Conditional analysis on the discovery cohorts ( Table 1 , Supplementary Fig. 4 ) showed additional independent signals at the TF locus for transferrin and transferrin saturation and at TMPRSS6 for iron. Gene-based analysis in the discovery cohort ( Supplementary Table 5 ) gave significant results (critical P -value for testing of 17,000 genes <3 × 10 −6 ) for ferritin in a region covering two genes ( C15orf43 and SORD ) on chromosome 15, where individual SNPs gave only suggestive associations. Allelic associations across this region are also shown in Supplementary Fig. 2 . This locus did not show any SNPs with genome-wide significance in the combined discovery+replication data. In the replication cohorts, the lead SNPs at the 11 significant loci explained 3.4, 7.2, 6.7 and 0.9% of the phenotypic variance for iron, transferrin, saturation and (log-transformed) ferritin, respectively. Allelic association results for all SNPs tested will be available from http://genepi.qimr.edu.au/ . Secondary analyses In view of the known association between ferritin concentration and inflammatory conditions, we repeated the discovery meta-analysis of ferritin including C-reactive protein (CRP, a marker of inflammation) as a covariate. This resulted in a decrease in effect sizes (expressed as standardized regression slopes or betas in an additive-allelic-effect model) for the lead SNPs at significant and suggestive loci, to an average of 73% (s.d. 15%) of the previous betas ( Supplementary Fig. 5 ). The P -values became less significant, partly because of the decrease in effect size and partly because the number of subjects with CRP data was less than the number available for the initial analysis. To check whether results were similar after excluding people with iron deficiency, we removed subjects with serum ferritin concentration below 30 μg l −1 and repeated the meta-analyses for all four phenotypes. This decreased effect sizes for transferrin and transferrin saturation, but had negligible effects for SNPs, which were significant or suggestive for ferritin or iron compared with those from the all-subjects analysis ( Supplementary Table 6 ). We also examined the association between serum transferrin concentration and FADS2 variation. Because this gene is known to be associated with other phenotypes related to lipids and components of the metabolic syndrome, we included high-density lipoprotein cholesterol (HDL-C) as a covariate and repeated the association meta-analysis for transferrin and the most significant SNP at the FADS2 locus, rs174577. (HDL-C was chosen because it was available for a greater proportion of subjects than either triglycerides or glucose, which are also associated with FADS polymorphisms.) This conditional analysis resulted in a 35% reduction in the effect size for this SNP, from β =0.068±0.011 to 0.044±0.009. Effects on gene expression and regulation We next checked for data that may help explain the biological role of the significant SNPs or identify the causal variants which they tag, using sources listed in Methods. The synthesis of information from our results and external sources is exemplified in Fig. 2 , which shows the alignment of data at the TFR2 locus. The region that includes genome-wide-significant SNPs (after replication) for serum iron contains documented eQTLs for TFR2 , and H3K27Ac histone modification sites (documented in data from ENCODE). In this case, there is striking alignment at the region around 100.2 Mbp at one end of the TFR2 gene, which includes the most significant SNPs at this locus, documented eQTLs for this gene, and the histone modification in K562 (erythroleukaemia) cells. 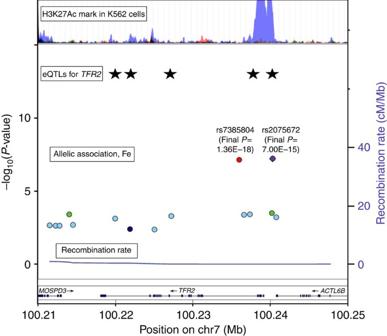Figure 2: Comparison of results for serum iron with regulatory features at the chromosome 7 (TFR2) locus. From bottom: regional association plot with recombination rate and −log(P) values for serum iron; documented eQTL locations forTFR2expression (from left to right: rs10247962, rs4729598, rs7457868, rs4729600, rs1052897); ENCODE data on histone modification.P-values for serum iron at rs7385804 and rs2075672 are shown as text (FinalP) for the Discovery+Replication dataset, but positions for all SNPs on theyaxis are determined by the Discovery dataset only. Figure 2: Comparison of results for serum iron with regulatory features at the chromosome 7 ( TFR2 ) locus. From bottom: regional association plot with recombination rate and −log( P ) values for serum iron; documented eQTL locations for TFR2 expression (from left to right: rs10247962, rs4729598, rs7457868, rs4729600, rs1052897); ENCODE data on histone modification. P -values for serum iron at rs7385804 and rs2075672 are shown as text (Final P ) for the Discovery+Replication dataset, but positions for all SNPs on the y axis are determined by the Discovery dataset only. Full size image A similar approach was taken for the other significant loci, as summarized in Supplementary Table 7 . SNPs identified through the GWAS had significant cis-effects on expression of SLC40A1 , TFRC , ARNTL and FADS1/FADS2 . At the C15orf43-SORD locus on chromosome 15, rs16976620 (allelic association with ferritin P =4.52 × 10 −7 ) affected expression of SORD at P =4.02 × 10 −4 . The chromosome 22 region near TMPRSS6 contains eQTLs for the hepatic expression of TMPRSS6 (ref. 24 ). However, the chromosome 3 locus near TF contains eQTLs for SRPRB but not for TF ; and SNPs at the loci identified as TFR2, ABO and TEX14 are eQTLs for multiple other genes. The ENCODE regulatory data show potential regulatory sequences or histone marks in the regions where we found SNP associations on chromosome 2 near SLC40A1 , chromosome 11 near the FADS genes, and at the chromosome 17 locus near TEX14 . Some lead SNPs from our significant loci also showed trans -effects on more distant genes ( Supplementary Table 7 ). Most notably, the three non-synonymous coding SNPs in HFE and TMPRSS6 (rs1800562, rs1799945 and rs855791) had strong effects on expression of ALAS2 (aminolevulinate, delta-, synthase 2), which catalyses the initial step in haem synthesis in erythroid tissues. Overlap with other phenotypes and disease associations Because of previous data showing that iron-related loci overlap with loci affecting erythrocyte phenotypes, and because several of our significant loci have been reported to affect lipid phenotypes, we compared our results against published meta-analysis data on erythrocytes and lipids. Results are summarized in Supplementary Table 8 . Among the 75 significant loci for erythrocyte phenotypes [25] , we found associations with one or more of our iron phenotypes after Bonferroni correction for multiple testing at P <6.7 × 10 −4 ( P <0.05 adjusted for testing of 75 SNPs) for ABO , HFE , TFR2 , TFRC and TMPRSS6 , and additionally for HBS1L ( P =9.78 × 10 −7 for transferrin saturation) and PGS1 ( P =1.84 × 10 −4 for ferritin). For the 157 lipid loci reported by the Global Lipids Genetics Consortium [26] , two loci ( HFE and HBS1L ) gave P <3.18 × 10 −4 ( P <0.05 adjusted for testing of 157 loci) for iron and saturation, six ( FADS1/2/3 , GCKR , HFE , NAT2 , SNX5 and TRIB1 ) for transferrin, and six ( ABO , HFE , LOC84931 , LRP1 , PGS1 and TRIB1 ) for ferritin. Moreover, plots of observed versus expected P -value distributions for the iron phenotypes ( Fig. 3 ) showed that even the erythrocyte and lipid loci not reaching statistical significance do affect iron biomarkers to a greater degree than can be explained by chance. 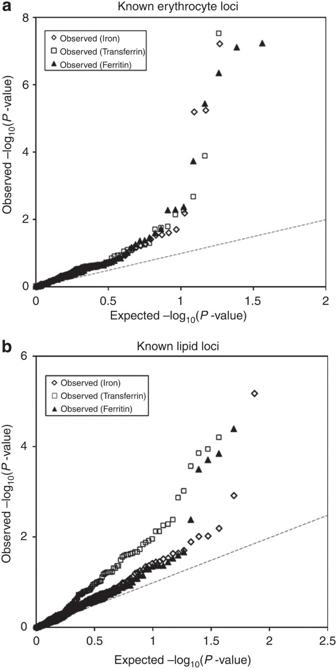Figure 3: Q–Q plots of the associationP-values for iron, transferrin and ferritin at loci previously reported to be significant for erythrocyte phenotypes25(upper panel, a) and plasma lipid phenotypes26(lower panel, b). For clarity, theyaxes only extend toP<10−8orP<10−6so that two associations with observedP<10−8for erythrocyte loci (atHFEandTMPRSS6) and four associations withP<10−6for lipid loci (atABO,FADS2,HFEandNAT2) are not plotted. The interrupted line in each plot is the line of equivalence, observed=expected. Figure 3: Q–Q plots of the association P -values for iron, transferrin and ferritin at loci previously reported to be significant for erythrocyte phenotypes [25] (upper panel, a) and plasma lipid phenotypes [26] (lower panel, b). For clarity, the y axes only extend to P <10 −8 or P <10 −6 so that two associations with observed P <10 −8 for erythrocyte loci (at HFE and TMPRSS6 ) and four associations with P <10 −6 for lipid loci (at ABO , FADS2 , HFE and NAT2 ) are not plotted. The interrupted line in each plot is the line of equivalence, observed=expected. Full size image The SNP association results were also analysed using Ingenuity Pathway Analysis, selecting SNPs, which showed associations at P <0.01, <0.001 and <0.0001 for transferrin saturation, and similarly for ferritin. Results for these two phenotypes, chosen as markers of iron availability and iron stores, showed substantial overlap. The P <0.01 threshold identified an excess of genes that have been reported to affect or be associated with lung cancer, cardiovascular disease and diabetes; and also with a range of developmental and nerve cell functions ( Supplementary Fig. 6 ). Results for the P <0.001 threshold were similar but showed lesser statistical significance, as expected because of the smaller number of genes included. Effects on iron status in HFE C282Y homozygotes We tested whether the lead SNPs at loci that affect iron-related biomarkers in the general population also explain variation in iron status in C282Y homozygotes who are at genetic risk of HFE -related iron overload. These comprised 76 homozygotes from the QIMR Adult cohort (one of the discovery cohorts), plus 277 homozygotes from the HEIRS study [27] . Results are shown in Table 2 for significant associations, and more fully in Supplementary Table 9 . Table 2 Results for HFE YY subjects. Full size table The strong association between rs8177240 in the TF gene and serum transferrin was clearly present in HFE YY homozygotes ( P =1.93 × 10 −9 ). The YY group showed association between serum iron and rs7385804 at TFR2 ( β =0.178±0.053, P =0.00076, critical P -value=0.005 after adjusting for testing of ten loci). The standardized beta for this SNP was approximately three times as great in the YY sample as in the overall meta-analysis (0.178±0.053 against 0.055±0.010). There was also a significant association ( P =0.0022) between rs6486121 in ARNTL and ferritin. When we checked for associations between a genetic risk score calculated from the significant and suggestive SNPs in the population-based meta-analysis results, and the biomarker phenotypes in the HEIRS sample, only transferrin showed a significant association and this was stronger among the men than the women ( Supplementary Table 10 ). Our meta-analysis of GWAS on iron-related phenotypes from up to 48,000 people of European descent showed multiple significant associations. Some increased the significance of loci known from previous studies or showed significant associations with additional phenotypes ( TF , TFR2 , HFE , TMPRSS6 ); some were at loci containing genes whose products have known roles in iron homeostasis, including the transferrin receptor TFRC and the iron transporter ferroportin ( SLC40A1 ); and others were novel (near to ARNTL , FADS2 and NAT2 for transferrin, ABO and TEX14 for ferritin). Significant associations were found for biomarkers of iron status that reflect both cellular iron metabolism and systemic regulation of iron [23] . There was variation in the phenotypes affected by the significant loci, as summarized in Supplementary Fig. 3 . Three of the loci mainly affected serum ferritin ( ABO , SLC40A1 , TEX14 ); three others mainly affected serum iron and transferrin saturation ( HFE , TFR2 , TMPRSS6 ); and five mainly affected serum transferrin ( ARNTL , FADS2 , NAT2 , TF and TFRC ). The loci with the strongest effects on serum iron ( HFE , TMPRSS6 ) had significant, but smaller, effects on serum ferritin and it is likely that this is due to higher circulating concentrations of iron leading over time to higher iron stores and hence higher serum ferritin. We note that there are factors that can modify the relationships between these biomarker phenotypes and whole-body or tissue-specific iron status. Ferritin has been criticized as a marker of iron stores because it is an acute-phase protein increased by inflammation, but comparisons with independent methods [28] , [29] have validated it sufficiently for use in epidemiological studies. Moreover, the loci that affected ferritin in this study have not been reported in GWAS for inflammatory biomarkers or CRP [30] , and SLC40A1 , which showed a highly significant association with ferritin, has strong biological plausibility because it codes for ferroportin. Including CRP as a covariate in the ferritin association analysis changed the effect size similarly for all the significant or suggestive SNPs ( Supplementary Fig. 5 ), whereas effects related to both inflammation and iron status would be expected to alter betas for some SNPs and not others. We also note that matching of significant loci to genes is subject to uncertainty. For some, the location of the peak association close to a gene with a known and relevant physiological function gives confidence in the gene assignment. For others, data from previous reports or databases on association between SNPs and gene expression will identify a probable gene, but in other cases expression data are consistent with any of several genes or else no relevant data are available. If so, the name of the nearest gene may be provided for identification of the locus but this may require revision as more information becomes available. Five confirmed loci contain genes ( TF , TFR2 , HFE , TMPRSS6 , SLC40A1 ) that were already known to affect iron homeostasis. These genes have been previously identified via monogenic diseases or from functional studies. Interestingly, no association has been identified with genes for several other important players in iron homeostasis such as ferritin, the protein that safely stores excess iron, or hepcidin and hemojuvelin, which are essential in the hepcidin signalling pathway and when mutated cause severe juvenile-onset hemochromatosis (type 2A, 2B). Mutations at the loci identified cause late-onset ( HFE , type 1) or less severe ( TFR2 , type 3 and SLC40A1 , type 4A) hemochromatosis. SNPs at HFE and TMPRSS6 that mainly affect iron and transferrin saturation showed interesting trans -effects on gene expression for ALAS2 . As this gene is on the X chromosome and we only analysed GWAS data for autosomes, we do not know whether ALAS2 variation affects our phenotypes. However, ALAS2 activity controls the initial and rate-limiting step in porphyrin synthesis so a co-ordinated effect on both iron and protoporphyrin availability for formation of haem is an interesting possibility. SLC40A1 is a prime candidate for affecting iron stores, as it codes for ferroportin and mutations in this gene are associated with the autosomal dominant type 4 hemochromatosis, characterized by high ferritin levels. The most significant SNPs near SLC40A1 in our study are about 45 and 60 kbp from the gene, but are known to affect SLC40A1 expression. Variation near SLC40A1 also affects transferrin, probably through an effect on cellular iron availability. Genome-wide studies of erythrocyte traits known to vary with iron status [20] , [21] , [22] , [25] have previously found associations with many of these loci: erythrocyte volume (MCV) and haemoglobin content (MCH) with HFE , TFR2 , TFRC and TMPRSS6; haematocrit with HFE , TFR2 , and TMPRSS6 ; and erythrocyte count with TFR2 (ref. 25 ). The results for our iron data at loci known to affect erythrocyte phenotypes are illustrated in Fig. 3a ; an unexpectedly high proportion of them affect iron, transferrin and ferritin. New associations were found for ferritin near ABO and TEX14 . The ABO blood group locus has shown significant associations for several phenotypes; rs651007 has a particularly strong effect on E-selectin [31] and has also been found in GWAS on low-density lipoprotein cholesterol [32] , coronary artery disease [33] and red blood cell count [25] . The latter is relevant to our ferritin finding, but whether ABO variation primarily affects iron stores and therefore erythrocyte count, or vice versa , is unclear. TEX14 codes for a testis-expressed protein, but there was no evidence for male–female heterogeneity in the effect on ferritin (p Het for the lead SNP, rs368243, was 0.45). The most significant SNPs are within the TEX14 gene but the suggestive-significance region extends across other genes. Expression data suggest that variation affecting RAD51C may be important, but the function of this gene (in DNA repair and meiosis) also has no obvious connection with iron status. The same holds for SEPT4 , for which rs411988 is an expression QTL. Another gene within the LD block, MTMR4 , deserves consideration because it changes SMAD phosphorylation, with possible effects on the BMP-SMAD pathway affecting control of hepcidin [34] . The region on chromosome 15 identified in the gene-based analysis is centred on C15orf43 but also overlaps with SORD (sorbitol dehydrogenase). SORD has no obvious connection with iron status and the function of the protein coded by C15orf43 is unknown, although there is some evidence that it is present in human plasma ( http://pax-db.org/#!protein/986968 , accessed 2014-03-27). These two loci illustrate the difficulty, which may be encountered in interpreting allelic associations; in some cases, the region containing the most significant results overlaps with several genes, there may be unrecognized regulatory regions with effects on more distant genes, and data on gene expression may not reflect expression in the relevant tissue. For all these reasons, assignment of significant effects to specific genes must often be provisional. Effects on transferrin were seen for most of the loci, which affect serum iron, including HFE , TF , TFRC , and TMPRSS6. Contrary to the result for TFRC , variation at the other transferrin receptor gene TFR2 did not affect transferrin concentration; this may reflect the different functions of the two receptors. TfRC is involved in cellular iron uptake, which may directly affect the regulation of transferrin expression. TfR2 on the other hand has been reported to be involved in hepatocyte sensing of circulating iron and signalling to hepcidin production, which may subsequently affect circulating levels of iron and the transferrin saturation. TfR2 variation could also affect these iron parameters through its effect on erythropoiesis [35] . Transferrin was also affected by SNPs near ARNTL , NAT2 and FADS2. The role of these in iron homeostasis is uncertain; transferrin is central to iron transport and receptor-mediated uptake by cells but these loci did not affect serum iron or ferritin. ARNTL , and its product BMAL1, is mainly known for interactions with CLOCK genes and generation of circadian rhythm. Notably, serum iron [16] , [36] , liver iron [37] , hepcidin [38] and TfR1 gene expression [39] all show circadian variation. The region affecting transferrin on chromosome 8 contains the NAT2 gene, which again has no obvious relevance for iron. It has been shown to affect lipids [32] and cardiovascular risk (see Supplementary Table 8 of ref. 40 ). The gene product is important for xenobiotic metabolism; NAT2 codes for an N -acetyl transferase, which determines fast- or slow-acetylator status. At FADS2 , the significant SNPs for transferrin are intronic but they affect expression of FADS genes. FADS1/2/3 variation affects a wide range of phenotypes including serum lipids [32] , [41] , polyunsaturated fatty acid content of serum phospholipids [42] ; fatty acid composition of membranes and phospholipids [43] ; fasting glucose and insulin response [44] , [45] and liver enzymes [46] . The most significant FADS SNPs for lipids are rs174546, rs174547 and rs174548 (refs 32 , 41 , 47 ) and each gave significant or near-significant P -values for transferrin in our data ( P =7.43 × 10 −10 , 8.47 × 10 −10 and 7.29 × 10 −8 , respectively). This, together with the decrease in the locus effect on transferrin after inclusion of HDL-C as a covariate, suggests a common basis for effects on lipids and transferrin. The pathways involved are unknown, but iron homeostasis and lipid metabolism show overlap in the literature [32] , [48] , [49] , [50] , [51] as well as in our data. It has recently been shown, for example, that signalling pathways for the protein kinase mTOR, which regulates energy metabolism and lipid synthesis among other functions [52] , affect transcriptional control of hepcidin and therefore potentially affect iron uptake and distribution [53] . Despite the varied functions of these three genes ( ARNTL , FADS2 , NAT2 ), which unexpectedly affect transferrin, they have the common feature of significant effects on plasma triglycerides [26] . Detailed comparison of our results against published lipid loci showed that a high proportion of lipid loci (not only for triglycerides) have detectable effects on our iron phenotypes, especially on transferrin ( Fig. 2b , Supplementary Table 8 ). The pleiotropic effects at such loci, connecting iron homeostasis not only with erythropoiesis but also with lipids and possibly with cardiovascular risk, deserve further investigation. One important clinical question about iron overload is why some HFE C282Y homozygotes develop biochemical evidence of iron overload and clinical symptoms of hemochromatosis, while most do not [54] . A systematic review of longitudinal studies found that 38–76% of homozygous people have increased ferritin and transferrin saturation (biochemical penetrance) [55] . However, clinical symptoms are less common at 2–38% in men and 1–10% in women [56] , [57] . We therefore evaluated the effects of our lead SNPs in HFE C282Y homozygotes, combining data from the largest of our Discovery cohorts with available phenotypic information and DNA from participants in the HEIRS study. Because of limited numbers of C282Y homozygotes (total N available for data analysis was 353), we had limited power to detect relevant effects. Among our results, the association between two SNPs in TFR2 and serum iron seems the most relevant. There is both clinical and experimental evidence for interaction between the gene products of HFE and TFR2 . Severe juvenile hemochromatosis occurred in a family carrying mutations in both HFE and TFR2 (ref. 58 ). In mice, homozygosity for deletion of both Hfe and TfR2 greatly decreases hepcidin levels [59] and causes massive iron overload [60] . These reports are consistent with evidence that TFR2 and HFE proteins interact in control of hepcidin signalling; they may form an iron-sensing complex that modulates hepcidin expression in response to blood levels of diferric transferrin [61] , [62] . Overall, there was a lack of correlation between effect sizes for lead SNPs at the significant loci identified in the general population, and in the YY homozygotes. Similarly, a predictor based on allele count and effect size for SNPs taken forward for replication and genotyped in the HEIRS subjects did not significantly predict iron, saturation or ferritin in the HEIRS C282Y homozygotes ( Supplementary Table 10 and Supplementary Fig. 7 ). The exception, transferrin, was due to the strong effects at the TF locus. Previous studies have proposed determinants of HFE clinical or biochemical penetrance. Apart from age, sex and probably alcohol intake [63] , the focus has been on genetic modifiers but no candidate has been convincingly identified [64] . Since iron homeostasis involves a complex regulating network [23] , [65] , it seems probable that any genetic effects on penetrance are either highly polygenic (in which case large genome-wide studies on HFE C282Y homozygotes will be needed) or result from rare variants, which have not yet been examined in sufficient detail. TFR2 variation as a modifier of HFE C282Y risk has statistical support and biological plausibility but confirmation is needed. Our results have revealed genes or loci whose effects on iron status were previously unsuspected and which need to be integrated into our understanding of iron homeostasis. Discovery of SNPs that significantly affect iron status, and compilation of genomic scores, will allow Mendelian randomization studies on the multiple conditions associated with variation in iron load and help to clarify a potential causal role of iron in such conditions (for example, Parkinson’s [14] or Alzheimer’s [66] diseases). However, the existence of pleiotropic effects, with many loci affecting both iron and lipid phenotypes, shows the need for caution in selecting SNPs or scores for such applications. Subjects We established the Genetics of Iron Status Consortium to coordinate our efforts in understanding the causes and consequences of genetic variation in biochemical markers for iron status, that is, serum iron, transferrin, transferrin saturation and ferritin. Discovery samples consisted of summary data on genome-wide allelic associations between SNP genotypes and iron markers from 23,986 subjects of European ancestry gathered from 11 cohorts in nine participating centres ( Supplementary Table 1 ). Replication samples to confirm suggestive and significant associations were obtained from up to 24,986 subjects of European ancestry in 8 additional cohorts (also in Supplementary Table 1 ). There was no systematic selection whether a cohort was allocated into the discovery or replication samples. This allocation was based on the availability of data when the analyses were conducted. Information on phenotypic means, methods for phenotype measurement, and genotyping methods for each contributing cohort are shown in Supplementary Tables 2 and 3 . Each participating study was approved by the appropriate human research ethics committee, as listed for each study in Supplementary Table 1 , and all subjects gave informed consent. GWAS Genome-wide association tests, genotype imputation and associated quality control procedures (QCs) were performed in each cohort separately. Within each cohort, QCs were applied to individual samples and SNPs before imputation into HAPMAP II (Release 22, NCBI Build36, dbSNP b126) or, for InterAct, 1,000 Genomes. These include removing individuals based on missingness, relatedness, population and ethnic outliers. Poor-quality SNPs were also removed based on missingness, minor allele frequency, Hardy–Weinberg equilibrium test and Mendelian errors for family data. These QCs for each cohort are summarized in Supplementary Table 3 . The association between genotyped and imputed SNPs and each iron phenotype was performed using an additive model for allelic effects, on the standardized residuals of the phenotype after adjusting for age, principal component scores and other study specific covariates, for each sex separately. The details of the association analysis and imputation method for each cohort are presented in Supplementary Table 3 . Meta-analysis We conducted meta-analysis of GWAS results from the discovery cohorts in the Metal package [67] using a standard error-based approach, which weights the SNP effect size (standardized regression slope, beta) using the inverse of the corresponding squared s.e. SNPs were included in the meta-analysis if they met the following conditions: imputation quality score either Rsq (which estimates the squared correlation between imputed and true genotypes) for MACH software ≥0.3, or the ‘info’ measure for IMPUTE software >0.5; Hardy–Weinberg Equilibrium Test P -value (pHWE) ≥10 −6 ; minor allele frequency ≥0.01; genotyping Call Rate ≥0.95 and if they survived QCs in all cohorts to avoid disproportionate contribution of a single cohort to the meta-analysis. In total, ~2.1 million SNPs met these conditions. A genomic control correction was applied to all cohorts. Heterogeneity of effect sizes between cohorts or between sexes was also assessed using Cochran’s Q statistic within Metal. Loci containing SNPs with P <5 × 10 −6 were carried forward for in silico replication in independent samples, again using Metal for the meta-analysis. The threshold P -value for choice of SNPs for replication is conventional and based in part on data for European populations in Duggal et al . [68] Power to detect allelic effects was estimated using the Genetic Power Calculator ( http://pngu.mgh.harvard.edu/~purcell/gpc/ ). Under reasonable assumptions about allele frequencies for causative and marker polymorphisms (QTL increaser allele frequency=0.2, marker allele frequency=0.2, linkage disequilibrium between them d ′=0.8, α =5 × 10 −8 ), the Discovery dataset with N =24,000 gives 77% power to detect allelic effects which each account for 0.25% of the phenotypic variance. Gene-based analysis Gene-based analysis considers all SNPs within a gene as a unit for the association analysis. We performed gene-based analysis on SNP association P -values from the meta-analysis of discovery samples using VEGAS ( http://gump.qimr.edu.au/VEGAS/ , accessed 2014-03-27) (ref. 69 ). The significance of gene-based analysis was based on Bonferroni correction of testing ~17,000 genes (that is, P <3 × 10 −6 ). Conditional analysis To find independent signals within each significant locus, we performed conditional analysis in each cohort by repeating the association analysis but including the most significant SNP at each significant locus (in the initial meta-analysis) as covariates. We performed meta-analysis of the conditional association results using the same approach as in the main meta-analysis. Gene expression The eQTL look-up was based on a meta-analysis of expression data for known disease-associated loci in non-transformed peripheral blood cells, from 5,300 samples from seven cohorts. The original analysis used HapMap2 imputed SNPs and a cis-window of ±250 kb from the transcription start-site. More details can be found in the paper by Westra et al . [70] Information on gene expression in macrophages and monocytes was based on results obtained by the Cardiogenics consortium, on 758 samples, as described in the Supplementary Note [33] . Online resources for gene expression and regulation included http://eqtl.uchicago.edu/cgi-bin/gbrowse/eqtl/ , http://genenetwork.nl/bloodeqtlbrowser/ and Schadt et al . [24] for eQTL data, http://genome.ucsc.edu/ENCODE/ for information on histone modification and http://ecrbrowser.dcode.org/ for comparison of DNA sequences across species. Bioinformatic analyses Pathway analysis and assessment of known disease associations or biological functions was performed using Ingenuity Pathway Analysis (IPA; Ingenuity Inc., Redwood City, CA, 94063), selecting SNPs, which showed associations at P <0.01,<0.001 and<0.0001 for transferrin saturation, and similarly for ferritin. IPA compares the list of genes associated with the selected SNPs against a proprietary library of gene-disease and gene-function associations and test frequencies of observed and expected occurrences. Analysis in HFE C282Y homozygotes Data and DNA samples from HFE C282Y homozygotes in the HEIRS study [27] were obtained from the NIH Biologic Specimen and Data Repository Information Coordinating Center ( BioLINCC ) ( https://biolincc.nhlbi.nih.gov/home/ ). HEIRS was a population-based survey of the prevalence and effects of HFE polymorphisms, and subjects were not selected for having a diagnosis or positive family history of hemochromatosis. Selected SNPs (those showing significant or suggestive results in our primary meta-analysis) were genotyped by primer-extension mass spectrometry (MassArray, Sequenom Inc, San Diego CA); all samples were confirmed as being homozygous for the minor allele of rs1800562 by this method. Allelic association results for the QIMR adults and HEIRS C282Y homozygotes were combined by meta-analysis. How to cite this article: Benyamin, B. et al . Novel loci affecting iron homeostasis and their effects in individuals at risk for hemochromatosis. Nat. Commun. 5:4926 doi: 10.1038/ncomms5926 (2014).